Tuning gap states at organic-metal interfaces via quantum size effects Organic-metal interfaces are key elements in organic-based electronics. The energy-level alignment between the metal Fermi level and the molecular orbital levels determines the injection barriers for the charge carriers at the interfaces, which are crucial for the performance of organic electronic devices. Dipole formation at the interfaces has been regarded as the main factor that affects the energy-level alignment. Several models have been proposed for the mechanism of dipole formation in the context of the interface between organic molecules and a bulk metal crystal surface, at which surface states were mostly used to probe the interfacial properties. Here we report that when the bulk metal crystal is replaced by a uniform metal thin film, the resulting two-dimensional quantum-well states will be able to not only probe but also modify the interfacial electronic structures, such as gap states, that have no counterpart at the organic-bulk crystal interface. Quantum confinement in a thin film [1] gives rise to discrete quantum-well states (QWS) and a thickness-dependent electronic structure. As a result, it can lead to dramatic atomic-layer-by-atomic-layer variations in physical properties such as the surface energy [2] , thermal stability [3] , work function [4] , superconducting-transition temperature [5] , [6] , electrical conductivity [7] and surface adsorption [8] , [9] . As for surface adsorption, most studies have been focused on the oxidization of thin films such as Mg [8] and Pb [9] , and oscillation of the surface oxidization rate with the thickness of such thin films has been observed. The physisorption of organic molecules on metal thin films has been studied by Lin et al. [10] , and from the thickness-dependent energy shift of Ag QWS, the dielectric constant of one-monolayer (ML) long-chain tetratetracontane (TTC) on the Ag films was extracted. In this paper, we report a systematical photoemission study of quantum size effects (QSE) on organic-metal interfaces by varying three factors: first, the thickness of the Ag films; second, the types of substrates for the Ag films, which are Ge(111), a semiconductor surface, and Au(111), a metal surface; and third, the types of adsorbates, which are mainly phthalocyanine-family molecules, such as copper phthalocyanine (CuPc), phthalocyanine (H 2 Pc) and tetra-tert-butyl H 2 Pc (TTB-H 2 Pc). In contrast to TTC, which is an insulator, phthalocyanine-family molecules are generally considered p -type electron donors. Therefore, a non-trivial interfacial electronic structure is expected with respect to the charge transfer as a result of the interaction between the molecular orbital state (MOS) and the Ag QWS in the context of chemisorption. Moreover, we discover that Ag QWS would carry the influence of the Ge substrate under the Ag film to the top organic-metal interface, as manifested by the QSE. 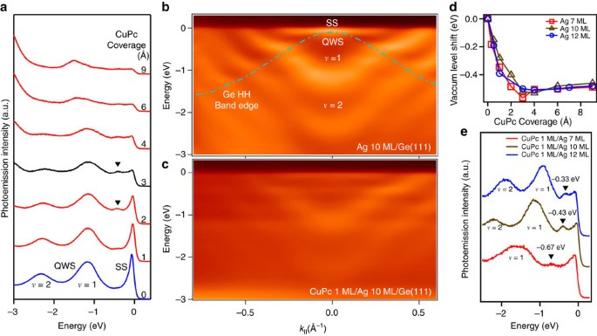Figure 1: Photoemission data for CuPc on Ag thin films on Ge(111). (a) Normal emission spectra as a function of CuPc coverage for 10-ML Ag thin film on Ge(111). (b) Angle-resolved photoemission result alongfor 10-ML Ag thin film on Ge(111). (c) Angle-resolved photoemission result alongfor 1-ML CuPc on 10-ML Ag thin film on Ge(111). (d) Vacuum-level shift as a function of CuPc coverage for 7-, 10- and 12-ML Ag thin films. (e) Normal emission spectra for 1-ML CuPc on 7-, 10- and 12-ML Ag thin films. The black wedges indicate the energy positions of the gap states. Angle-resolved photoemission spectroscopy Figure 1a shows energy-distribution curves (EDCs) at normal emission for increasing CuPc on 10-ML Ag film/Ge(111). As observed, the peak intensities of the Ag surface state (SS) near the Fermi level and the QWS attenuate as the CuPc coverage increases. However, at a CuPc coverage of ~1 Å, there is evidence of a peak emerging at an energy of −0.43 eV and, subsequently, it saturates in intensity at a coverage of 3 Å. On further adsorption, this peak as well as the Ag QWS and SS peaks diminish, and the CuPc highest occupied molecule orbital (HOMO) peak shows up at approximately −1.5 eV. This anomalous peak should be related to the interface, and because it is located between the CuPc HOMO and lowest unoccupied molecule orbital (LUMO) levels, it should be a gap state. Figure 1b show the two-dimensional (2D) photoemission spectra of energy-band dispersions for 10-ML Ag film/Ge(111) and 3 Å CuPc coverage on 10-ML Ag film/Ge(111), respectively, in the symmetry direction from . According to previous work regarding the QWS electronic structures of uniform Ag films grown on Ge(111) [11] , the bulk band edges of Ge, namely, heavy hole (HH), light hole (LH), and split-off (SO), would have Anderson-type electron–electron interactions with Ag QWS, causing a distortion or kink of the QWS dispersion at the intersection point with the Ge band edges, among which the HH band edge, which is depicted by the dash-dotted curve in Fig. 1b , exhibits the strongest effect. It is of note that the parts of the QWS bands that are observed below the Ge HH band edge are resonances because they overlap with the bulk Ge continuum. The band of the gap state observed in Fig. 1a is found to be flat at the energy position (−0.43 eV) that corresponds to the top edge of the kink where the QWS band ( v =1) and the Ge HH band cross each other, as shown in Fig. 1c . Hence, it is seemingly implied that this gap state is related to the Ge substrate under the Ag films. Another flat band observed at approximately −1.25 eV is derived from the HOMO state for the first-layer CuPc on Ag(111) [12] . Figure 1d shows the vacuum-level shifts as a function of CuPc coverage on Ag films of 7, 10 and 12 ML; all exhibit similar decreasing trends with increasing coverage and begin to saturate at ~3 Å. We therefore set the coverage of 3 Å to correspond to one ML for CuPc. The Ag-thickness dependence of this gap state at a CuPc coverage of one ML was further examined; as shown in Fig. 1e , as the Ag thickness increases, the gap state shifts in energy towards the Fermi level with increasing peak intensity and decreasing line width. The energy positions of the gap state at Ag thicknesses of 7 ML and 12 ML are −0.67 and −0.33 eV, respectively; the QSE of the Ag films on the interfacial electronic structures of the CuPc-Ag interface is evident. The dependence of the gap-state energy on the Ag-film thickness can be understood from the fact that the gap state occurs at the crossing point between the QWS band and the Ge band edge, which must change, as the entire QWS band shifts in energy with varying Ag thickness. Figure 1: Photoemission data for CuPc on Ag thin films on Ge(111). ( a ) Normal emission spectra as a function of CuPc coverage for 10-ML Ag thin film on Ge(111). ( b ) Angle-resolved photoemission result along for 10-ML Ag thin film on Ge(111). ( c ) Angle-resolved photoemission result along for 1-ML CuPc on 10-ML Ag thin film on Ge(111). ( d ) Vacuum-level shift as a function of CuPc coverage for 7-, 10- and 12-ML Ag thin films. ( e ) Normal emission spectra for 1-ML CuPc on 7-, 10- and 12-ML Ag thin films. The black wedges indicate the energy positions of the gap states. Full size image As it was speculated that the Ge(111) substrate was involved in the formation of the observed gap state, we further investigated the system of CuPc deposited on Ag films/Au(111), which, in contrast to Ag films/Ge(111), has a small lattice mismatch (~1%) [13] , which leads to a negligible reflectivity at the interface, and hence quantum-well resonances partially confined within the Ag films should be less likely to exist [13] , [14] , [15] . 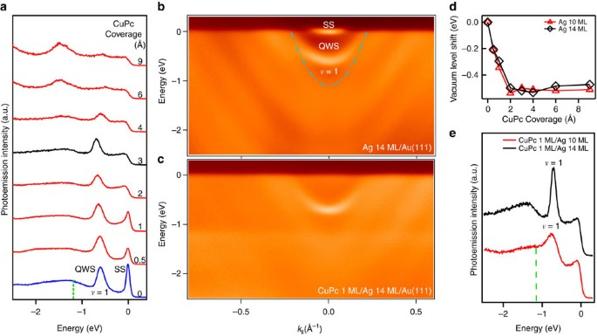Figure 2: Photoemission data for CuPc on Ag thin films on Au(111). (a) Normal emission spectra as a function of CuPc coverage for 14-ML Ag thin film on Au(111). (b) Angle-resolved photoemission result alongfor 14-ML Ag thin film on Au(111). (c) Angle-resolved photoemission result alongfor 1-ML CuPc on 14-ML Ag thin film on Au(111). (d) Vacuum-level shift as a function of CuPc coverage for 10- and 14-ML Ag thin films. (e) Normal emission spectra for 1-ML CuPc on 10- and 14-ML Ag thin films. The green dashed line indicates the L edge of the projected bulk band of Au. Figure 2a shows EDCs at normal emission for increasing CuPc coverage on 14-ML Ag film/Au(111). As demonstrated here, only the QWS at an energy higher than the Au bulk L -gap edge approximately −1.09 eV ( [14] ) exists, indicating that it corresponds to a fully confined state within the Ag film. Similar to the former case, the peak intensities of the Ag SS near the Fermi level and the QWS also attenuate as the CuPc coverage increases. However, the corresponding gap state is not observed throughout the entire range of CuPc coverage in Fig. 2a . Figure 2b show the 2D photoemission spectra of energy-band dispersions for 14-ML Ag film/Au(111) and 3 Å CuPc coverage on 14-ML Ag film/Au(111), respectively, in the symmetry direction from . The dash-dotted curve in Fig. 2b depicts the Au bulk band edge projected onto the (111) surface. The QWS observed in Fig. 2a exhibits a free-electron-like dispersion within the gap, completely different from the case for Ag films on Ge(111), in which the Ag QWS dispersions are distorted because of the interaction with the Ge bulk band edges. Consequently, the flat band of the gap state in the former case is not observed in Fig. 2c , except for the flat band that corresponds to the first-layer HOMO state at approximately −1.25 eV. As shown in Fig. 2d , the vacuum-level shifts of 10-ML and 14-ML Ag films/Au(111) on adsorption of CuPc are similar to those for Ag films/Ge(111) in the sense that they decrease and saturate at approximately −0.5 eV. Figure 2e shows the EDCs of the same energy range as those in Fig. 1e for Ag films of 10 and 14 ML on Au(111); again, no corresponding gap states are observed. Figure 2: Photoemission data for CuPc on Ag thin films on Au(111). ( a ) Normal emission spectra as a function of CuPc coverage for 14-ML Ag thin film on Au(111). ( b ) Angle-resolved photoemission result along for 14-ML Ag thin film on Au(111). ( c ) Angle-resolved photoemission result along for 1-ML CuPc on 14-ML Ag thin film on Au(111). ( d ) Vacuum-level shift as a function of CuPc coverage for 10- and 14-ML Ag thin films. ( e ) Normal emission spectra for 1-ML CuPc on 10- and 14-ML Ag thin films. The green dashed line indicates the L edge of the projected bulk band of Au. Full size image Therefore, a very intriguing and novel picture appears: the bottom Ge substrate underneath Ag thin films can affect the interfacial electronic structures between the top CuPc molecules and the Ag thin films via the interactions mediated by QWS. However, before further investigating this picture, we would like to understand how this special gap state is related to adsorbates. 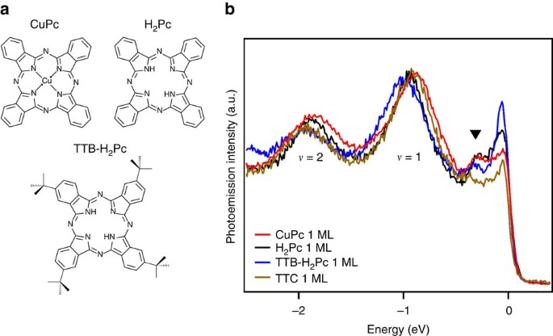Figure 3: Experimental evidence for the origin of the gap state. (a) Chemical formula of the CuPc, H2Pc and TTB-H2Pc molecules. (b) Normal emission spectra for 1-ML CuPc, H2Pc, TTB-H2Pc, and TTC on 12-ML Ag thin films/Ge(111). Figure 3a displays the chemical structures of three phthalocyanine-family molecules: CuPc, H 2 Pc and TTB-H 2 Pc. Two possibilities must be examined carefully. First, is this gap state derived from the charge transfer between the centred copper atom and the Ag films? Second, is this gap state related to the major components of the molecules, aromatic rings, that have π -bond electrons? As shown in Fig. 3a , H 2 Pc lacks the centred metal atom and TTB-H 2 Pc has four TTB substitutions on the periphery of H 2 Pc; thus, the entire H 2 Pc molecule and the aromatic rings would be slightly lifted above the Ag surface. In Fig. 3b , for the sake of comparison, we present together the EDCs at normal emission for 1 ML of CuPc, H 2 Pc, TTB-H 2 Pc and TTC on 12-ML Ag film/Ge(111). As can be observed, the gap states are of high intensity for CuPc and H 2 Pc but low intensity for TTB-H 2 Pc. TTC, which has mainly σ -bonding characteristics for alkane long-chain molecules, exhibits negligible intensity of the gap state. Therefore, the crucial role of π -bond electrons in aromatic rings for the formation of the observed gap state is confirmed. Figure 3: Experimental evidence for the origin of the gap state. ( a ) Chemical formula of the CuPc, H 2 Pc and TTB-H 2 Pc molecules. ( b ) Normal emission spectra for 1-ML CuPc, H 2 Pc, TTB-H 2 Pc, and TTC on 12-ML Ag thin films/Ge(111). Full size image Model explanation The energy positions of the gap states are observed to be at the top edge of the kink where the QWS band and Ge HH band edge cross each other; the density of states (DOS) of the QWS band would correspondingly exhibit a dramatic change at this energy because of the distorted curvature of the kink. For a 2D electronic system, the DOS is related to the energy-band curvature, namely, , by the relation where m* , which is equivalent to , and E 0 are the effective mass and the onset energy of the 2D electronic band, respectively. k is the magnitude of the wave vector parallel to the surface. We thus extract the DOS of the QWS band as a function of energy via the band curvatures. As shown in Fig. 4a for the 2D energy-band dispersion of 12-ML Ag film on Ge(111), the corresponding DOS for the QWS band of v =1 is depicted by the curve on the right-hand side of the energy axis. It is apparent that the DOS undergoes an abrupt increase throughout the energies near the kink because of the sharp curvature change of its top (higher peak) and bottom (lower peak) edges. The bottom edge of the kink belongs to the resonance with part of the charge density within the bulk Ge; thus, only the effect of the top edge is considered because it belongs to QWS fully confined within the Ag thin films and thus certainly has a much higher probability of interacting with the top adsorbates. For the 12-ML Ag film, supposedly, there should be 12 QWS subbands crossing the Ge HH band edge, causing 12 kinks in one symmetry direction. However, we focus on the top edge of the kink of the topmost ( v =1) QWS because only the flat gap-state band at this position is observed because of its proximity to the Ge gap above the HH band edge, which preserves a long lifetime of the electron states within it. We built the total DOS for all QWS subbands by summing the contributions from each QWS subband using equation (1). The onset energy positions of the 12 QWS subbands at normal emission, namely, E 0 , were obtained via the Bohr–Sommerfeld quantization rule using the phase-shift function at the Ag–Ge interface that was extracted from the measured QWS energy positions [16] , and the corresponding effective masses were acquired using equation (5) in [16] . As shown in Fig. 4b , in addition to the step-like DOS ascribed to each QWS subband, we imposed a delta-function-like peak at the energy position −0.33 eV to represent the effect caused by the kink of the ( v =1) QWS band. 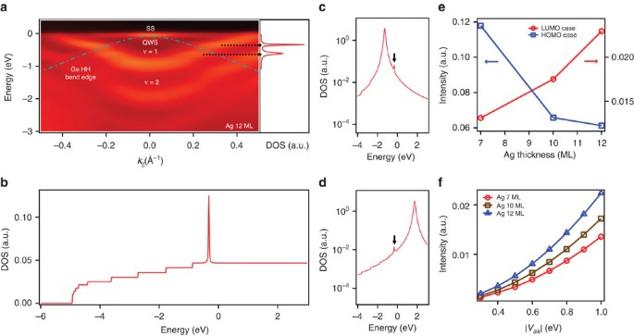Figure 4: Theoretical evidence for the origin of the gap state. (a) Left panel: the angle-resolved photoemission spectra for 12-ML Ag thin film on Ge(111) along. Right panel: the extracted DOS at the region where the Ge HH band edge crosses the QWS band. (b) Extracted DOS including contributions from all subbands of the QWS. (c) Projected DOS (in log scale) induced by the interaction between the pristine CuPc HOMO state and the QWS bands. (d) Projected DOS (in log scale) induced by the interaction between the pristine CuPc LUMO state and the QWS bands. (e) Intensities of the LUMO-induced states and the HOMO-induced states versus Ag thickness. (f) Intensities of the LUMO-induced gap states as a function of the interaction matrix element. Subsequently, the Newns–Anderson model for the chemical adsorption of an atom on a bulk metal surface [17] , [18] , [19] Figure 4: Theoretical evidence for the origin of the gap state. ( a ) Left panel: the angle-resolved photoemission spectra for 12-ML Ag thin film on Ge(111) along . Right panel: the extracted DOS at the region where the Ge HH band edge crosses the QWS band. ( b ) Extracted DOS including contributions from all subbands of the QWS. ( c ) Projected DOS (in log scale) induced by the interaction between the pristine CuPc HOMO state and the QWS bands. ( d ) Projected DOS (in log scale) induced by the interaction between the pristine CuPc LUMO state and the QWS bands. ( e ) Intensities of the LUMO-induced states and the HOMO-induced states versus Ag thickness. ( f ) Intensities of the LUMO-induced gap states as a function of the interaction matrix element. Full size image was employed to simulate the DOS resulting from the interaction between the Ag QWS and the CuPc MOS. In this model, ε a and n a represent the energy position of the single state before adsorption and the projected DOS after adsorption, respectively. Δ and Λ represent the imaginary and real parts, respectively, of the self-energy for the many-body interaction between the single state and the metal bulk continuum, whose DOS, n k ( ε ), typically exhibits a smooth dependence. In the case of the bulk sp band, which possesses a large bandwidth, the imaginary part of the self-energy, Δ, can be approximated by the relation [17] where | V ak | is the matrix element for the interaction, which can be considered to be a constant when | V ak | is much less than the bandwidth. The real part of the self-energy, Λ, is then derived from the imaginary part using the Kramers–Kronig relations. For our purpose, the smooth -dependent DOS, n k ( ε ), was replaced by that shown in Fig. 4b , and the HOMO and LUMO energies for the first layer of CuPc, −1.25 eV ( [12] ) and 1.75 eV, respectively, were used for ε a in light of the LUMO–HOMO gap of ~3 eV ( [20] ). With | V ak | reasonably set to 0.8 eV, as shown in Fig. 4c , the resulting projected DOS, n a ( ε ), exhibits a small but sharp peak, indicated by arrows, at exactly the same energy position as that of the top edge of the kink, −0.33 eV, in addition to the intense peaks that correspond to the HOMO and LUMO states after adsorption. Needless to say, this sharp peak indicates the observed gap state. We performed the same simulation for CuPc on 7- and 10-ML Ag film/Ge(111), and the intensity of the induced peak was found to be proportional to the Ag thickness for the case of the LUMO interacting with the Ag film, as opposed to the case for the HOMO ( Fig. 4e ). Note that this behaviour is consistent with that shown in Fig. 1e and, therefore, we can reason that the observed gap state is induced by the interaction between the CuPc LUMO and the QWS of the Ag thin films. Another simulation, shown in Fig. 4f , demonstrates the proportionality of the induced peak intensity to the value of the interaction matrix element, which connects the wave functions of the MOS and the Ag QWS. The π -bond electron of an aromatic ring is of p z type, as is the Ag QWS derived from the Ag bulk band from Γ to L, perpendicular to the (111) surface [13] . Therefore, the same symmetry of the two wave functions would lead to the maximum value of the interaction matrix element; on the contrary, a TTC molecule, which has a mainly σ -bonding character, adsorbed on an Ag film/Ge(111) would exhibit a reduced value of the interaction matrix element in terms of symmetry parity, thus leading to the negligible intensity of the gap state, as shown in Fig. 3b . As observed in Fig. 1e , the gap state for CuPc on 12-ML Ag film/Ge(111) is most intense and closest to the Fermi level; therefore, its impact on the energy-level alignment (ELA) between the energy levels of the CuPc and the Ag films should be most relevant. 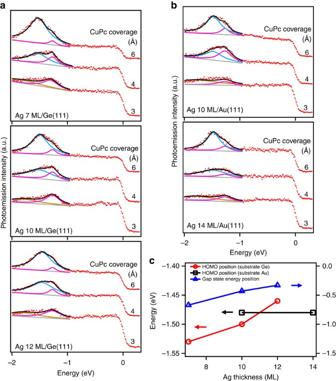Figure 5: The impact of the gap state on ELA. (a) The line shapes of the HOMO states for 3-, 4- and 6-Å CuPc on 7-, 10- and 12-ML Ag thin films on Ge(111). (b) The line shapes of the HOMO states for 3-, 4- and 6-Å CuPc on 10- and 14-ML Ag thin films on Au(111). The red dots represent the raw data. The dark curve represents the fitting result. The pink and blue curves represent the components of the first- and second-layer HOMO states for CuPc, respectively. The brown and grey curves represent the SO state at the submonolayer regime of CuPc and the background, respectively. (c) The dependence of the energy positions of the gap state and the second-layer HOMO on the Ag thickness for Ag thin films on Ge(111) and Au(111). Figure 5a shows the coverage-dependent EDCs of the HOMO states at an off-normal position ( k =0.8 Å −1 ), where the interference from the Ag QWS bands is negligible; hence, their intrinsic line shapes are suitable to reveal the layer resolution of the CuPc films. We fit the HOMO line shapes, taking into account the components of the SO state fixed at −1.75 eV ( [12] ) and the first and second CuPc layers [12] . For Ag thicknesses of 7, 10 and 12 ML, the first-layer HOMO positions are approximately the same, −1.27 eV, which is very close to the value of −1.25 eV measured for CuPc on a bulk Ag(111) crystal surface [12] . Neither the HOMO energy of the first-layer CuPc nor the SO state undergoes a noticeable shift with varying Ag thickness, possibly because the density of gap state (DGS) is not sufficient to have an impact on the ELA. With increasing coverage, the component of the HOMO line shape for the second layer emerges, but at different energies for different Ag thicknesses, that is, −1.53 eV for 7 ML, −1.50 eV for 10 ML and −1.46 eV for 12 ML. Note that −1.53 eV is also similar to its counterpart, −1.56 eV, for CuPc on bulk Ag(111) [12] . Figure 5b depicts the same analysis for CuPc on 10-ML and 14-ML Ag films/Au(111), which do not have the corresponding gap states, and the result indicates that the energy positions of the first-layer and second-layer CuPc, −1.27 and −1.48 eV ( [21] ), respectively, are the same for both Ag films, reflecting the effect of the gap state on the ELA for CuPc/Ag films/Ge(111). Unlike CuPc on Ag films/Ge(111), the second-layer HOMO bands of CuPc on 10- and 14-ML Ag films/Au(111) actually exhibit slight dispersion. The value −1.48 eV was measured at k =0.8 Å −1 , but at the surface zone centre ( k =0 Å −1 ) the energy position of the second-layer HOMO for both cases is −1.53 eV. Figure 5c reorganizes the dependence of the gap states and the second-layer HOMO positions on the Ag-film thickness for CuPc/Ag films/Ge(111) and CuPc/Ag films/Au(111). A previous study of the absorption of thin CuPc layers on bulk Ag(111) [12] has discovered a very weak and broad gap state, called the partially filled LUMO, at −0.15 eV, which was ascribed to the charge transfer from the Ag Fermi level to the CuPc LUMO. This explanation is consistent with our argument, derived from the simulation in Fig. 4e , that the observed gap state is induced by the interaction between the Ag QWS and the CuPc LUMO. As mentioned earlier, CuPc is a p -type electron donor with a smaller work function than that of Ag. On initial contact, charges would transfer from CuPc to Ag, thereby lowering the initial CuPc Fermi level and the LUMO and HOMO positions. However, the back donation of the charge from Ag to CuPc via the gap state would limit the lowering of the CuPc energy levels such that the actual HOMO position is closer to the Ag Fermi level with increasing DGS at the Ag Femi level, and exactly this phenomenon is manifested by the triangles and circles in Fig. 5c . The work presented here correlates the DOS of metal thin films and pinning position qualitatively via the Newns–Anderson model, whereas the quantitative relation will acquire the precise determination of the DOS, which is beyond the simple configuration depicted in Fig. 4b . Figure 5: The impact of the gap state on ELA. ( a ) The line shapes of the HOMO states for 3-, 4- and 6-Å CuPc on 7-, 10- and 12-ML Ag thin films on Ge(111). ( b ) The line shapes of the HOMO states for 3-, 4- and 6-Å CuPc on 10- and 14-ML Ag thin films on Au(111). The red dots represent the raw data. The dark curve represents the fitting result. The pink and blue curves represent the components of the first- and second-layer HOMO states for CuPc, respectively. The brown and grey curves represent the SO state at the submonolayer regime of CuPc and the background, respectively. ( c ) The dependence of the energy positions of the gap state and the second-layer HOMO on the Ag thickness for Ag thin films on Ge(111) and Au(111). Full size image The gap state [21] , [22] , an interfacial electronic structure, could greatly improve the hole injection for organic devices such as organic light-emitting devices [23] but could also, in contrast, reduce the efficiency of electron-hole formation for solar-cell devices [24] . Therefore, an effective method of tuning the gap state for the best device performance is very crucial. This paper demonstrates that by adjusting the integer thickness of the uniform Ag films underneath the CuPc molecules, the energy position of the induced gap state, which is derived from the kink of the Ag QWS band due to its strong interaction with the Ge bulk band edge, can be changed with respect to the Ag Fermi level, consequently causing a change in the ELA. A similar gap state, the partially filled LUMO, has been observed for CuPc on a bulk Ag(111) surface [12] . However, once the bulk is replaced by a uniform thin film, the QSE causes the gap-state energy to be tunable, and the sharp curvature change at the kink of the QWS band further enhances the DGS compared with that for CuPc on bulk Ag, leading to a greater impact on device function. On the other hand, from the scientific point of view, our result also illustrates that the role of the QWS is similar to the case of a non-magnetic metal thin film sandwiched between the top and the bottom magnetic films [25] , [26] , in which the QWS of the middle thin film dictate the spin coupling between the two magnetic films. The interaction between the Ag QWS bands and the Ge bulk band edges has been proven to be a two-dimensional-to-three-dimensional Anderson interaction [11] , and the chemisorption of CuPc molecules on Ag thin films can be observed as a zero-dimensional-to-two-dimensional version of the same interaction. Apparently, the observed induced gap state is the product of an indirect zero-dimensional-to-three-dimensional Anderson interaction mediated by the Ag QWS between the top organic molecules and the bottom Ge substrate. Such behaviour in terms of Anderson interaction is newly observed and of scientific interest. Photoemission measurements Angle-resolved photoemission spectra were collected using the commercial energy analyser Scienta R3000. The photoemission experiments were performed using a photon energy of 50 eV at the BL08-Al beamline at the National Synchrotron Radiation Research Center in Taiwan. The energy resolution of our system is ~50 meV. Sample preparation Here, n -type doped Ge(111) wafers and Au(111) crystal were chosen as the substrates. Through the standard sputtering and annealing processes, clean surfaces of Ge(111)-c(2 × 8) and Au(111)- × 22 reconstruction were obtained. Afterwards, the substrate was cooled to −140 °C for Ag deposition, followed by mild annealing at room temperature to form uniform Ag thin films. The organic molecules (CuPc, H2Pc and TTB-H2Pc) were then evaporated using Knudsen cells onto Ag films at room temperature, and the coverage of the organic films was monitored using a thickness monitor. How to cite this article: Lin, M.-K. et al. Tuning gap states at organic-metal interfaces via quantum size effects. Nat. Commun. 4:2925 doi: 10.1038/ncomms3925 (2013).